Cell death versus cell survival instructed by supramolecular cohesion of nanostructures Many naturally occurring peptides containing cationic and hydrophobic domains have evolved to interact with mammalian cell membranes and have been incorporated into materials for non-viral gene delivery, cancer therapy or treatment of microbial infections. Their electrostatic attraction to the negatively charged cell surface and hydrophobic interactions with the membrane lipids enable intracellular delivery or cell lysis. Although the effects of hydrophobicity and cationic charge of soluble molecules on the cell membrane are well known, the interactions between materials with these molecular features and cells remain poorly understood. Here we report that varying the cohesive forces within nanofibres of supramolecular materials with nearly identical cationic and hydrophobic structure instruct cell death or cell survival. Weak intermolecular bonds promote cell death through disruption of lipid membranes, while materials reinforced by hydrogen bonds support cell viability. These findings provide new strategies to design biomaterials that interact with the cell membrane. Nature utilizes amphiphilic peptides and proteins for a diverse set of functions including self-defence and vesicular trafficking [1] , [2] . The cationic and hydrophobic domains of these molecules enable them to associate strongly with cell membranes, often resulting in their disruption [3] , [4] , [5] , [6] . The two main classes of these membrane-permeable peptides, cell penetrating peptides and natural host defence peptides, have shown efficacy in a variety of applications including cancer therapy, antimicrobials, immune adjuvant therapy and delivery of genes, drugs or proteins [4] , [7] , [8] , [9] , [10] , [11] . These studies, however, typically evaluate the function of these peptides in solution. With an increasing interest in immobilizing functional peptides to multi-functional nanocarriers or nanostructured materials, there is great need to understand the interactions between cell membranes and materials rather than just molecules containing hydrophobic and cationic domains. Self-assembling peptide-based materials have gained recent attention because of their biocompatibility and widespread potential in biological applications [10] , [12] , [13] , [14] , [15] . Peptide materials can also be designed to utilize intermolecular interactions to form supramolecular nanostructures of various shapes, particularly high-aspect ratio nanofibres that emulate components of the mammalian extracellular matrix [14] , [15] , [16] , [17] , [18] . Among these self-assembling systems are peptide amphiphiles (PAs), a class of molecules containing an alkyl tail covalently attached to the end of a peptide chain [14] . Modifying the amino-acid sequence and extent of hydrogen bonding among PA molecules drastically affects the shape of their supramolecular assemblies and their ability to form three-dimensional networks [19] , [20] , [21] . Recent studies have also demonstrated that altering hydrogen bonding and electrostatic forces in these assemblies can directly control the stiffness of the materials they form and their ability to signal cells [22] , [23] , [24] . In this work, we investigate the influence of hydrogen bonding, hydrophobic domains and charge of PA materials on their interactions with cells. We demonstrate that the intermolecular interactions within nanostructures, particularly hydrogen bonding, influences cell viability and membrane integrity. Less cohesive assemblies rapidly associate with the phospholipid bilayer, causing disruption of the cell membrane and contact-mediated cell death. Interestingly, we find that materials that instruct cell death can be used to create a barrier to cell migration in 3D cultures. On the other hand, cell viability is rescued by increasing intermolecular interactions within the nanostructures. These interactions may play a role in the toxicity of naturally occurring biological assemblies, and can be used as a design criterion for nanostructured biomaterials for effective cell signalling or delivery of cargo. Linking supramolecular cohesion with cytotoxicity Many PA materials promote cell survival and elicit specific cell responses such as adhesion, proliferation and differentiation; however, the assemblies in this work demonstrate striking differences in cell viability. We systematically varied basic structural components of a model PA molecule PA 1 ( Fig. 1a , PA variations: Supplementary Fig. 1 ) to explore the role of hydrophobic collapse, charge and intermolecular forces on assembly morphology and cell response. Cells were cultured on PA-coated surfaces to provide a defined interface where cell–material contact could be visualized. Their viability was evaluated by fluorescent LIVE/DEAD staining, which was confirmed by measuring release of the ubiquitous, cytoplasmic enzyme lactate dehydrogenase (LDH) in the culture medium ( Fig. 1d ). 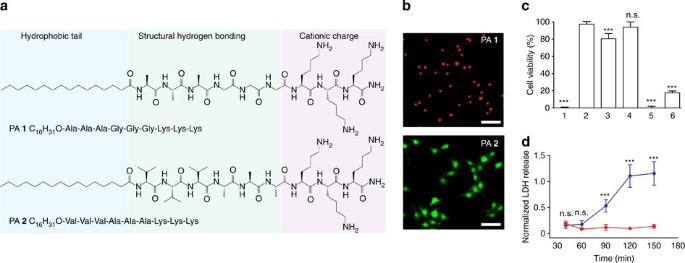Figure 1: Design of membrane-interacting self-assembling molecules. (a) Chemical structures of PA1and PA2that conserve the alkyl tail length (hydrophobic tail) and the number of lysine residues (cationic charge) but vary the propensity for intermolecular hydrogen bonding adjacent to the tail. (b) Representative fluorescence images of MC3T3-E1 cells that are viable (green, calcein) or dead (red, EthD-1) on coatings of each PA after 4 h of culture. Scale bars, 100 μm. (c) Quantification of cell viability from MC3T3-E1 cells on each PA coating including PAs3–6that vary the alkyl tail length and number of lysine residues (Supplementary Fig. 2). One-way ANOVA with Tukey post-test, ***P<0.001, compared with PA2. (d) LDH release over time of cells seeded on coatings of either PA1(blue) or PA2(red). Two-way ANOVA with Bonferroni post-test, ***P≤0.001. Figure 1: Design of membrane-interacting self-assembling molecules. ( a ) Chemical structures of PA 1 and PA 2 that conserve the alkyl tail length (hydrophobic tail) and the number of lysine residues (cationic charge) but vary the propensity for intermolecular hydrogen bonding adjacent to the tail. ( b ) Representative fluorescence images of MC3T3-E1 cells that are viable (green, calcein) or dead (red, EthD-1) on coatings of each PA after 4 h of culture. Scale bars, 100 μm. ( c ) Quantification of cell viability from MC3T3-E1 cells on each PA coating including PAs 3 – 6 that vary the alkyl tail length and number of lysine residues ( Supplementary Fig. 2 ). One-way ANOVA with Tukey post-test, *** P <0.001, compared with PA 2 . ( d ) LDH release over time of cells seeded on coatings of either PA 1 (blue) or PA 2 (red). Two-way ANOVA with Bonferroni post-test, *** P ≤0.001. Full size image PA 1 demonstrated strong cytotoxicity and rapid cell death ( Fig. 1b–d ) and provided a foundation for molecular design from which rescue could be assessed. The hydrophobic tail and cationic charge were essential for cell toxicity, as both the peptide sequences alone and the anionic analogue of PA 1 were found to be non-toxic ( Supplementary Fig. 2 ). We speculate that the non-toxic nature of the anionic PA is due to electrostatic repulsion, as the cell surface carries a negative charge due to the presence of glycoproteins and polysaccharide chains. Furthermore, reducing the amphiphilic nature of the assemblies by decreasing the alkyl tail length from 16 to 12 carbons or removing one lysine residue both supported cell viability (PA 4 , PA 3 , Supplementary Fig. 1 ). Concurrent with reducing toxicity, shortening the tail length also resulted in a shape change. A similar observation was reported by researchers that reduced the hydrophobicity of an amphiphilic, lysine-bearing peptide and found that a reduction in hydrophobicity correlated with less disruption of lipid membranes and a change in assembly morphology [25] . Furthermore, the trend in toxicity with reducing overall charge of the PA assemblies is consistent with previous reports, where reducing the overall cationic charge of amphiphilic molecules resulted in less cytotoxicity [26] . Although hydrophobicity and cationic charge influence the cytotoxicity of PA assemblies, the most striking difference was observed when modifying β-sheet hydrogen bonding among molecules within the nanostructure. A fibrous structure was observed in solution ( Fig. 2a ) and in coatings ( Supplementary Fig. 3 ) for both PA 1 and PA 2 , although they differ in amino-acid composition. PA 1 contains glycine and PA 2 valine, which has a higher propensity for β-sheet hydrogen bonding [27] , [28] . Interestingly, the cell toxicity was abolished when cells were exposed to PA 2 nanofibre coatings as indicated by viability staining and the lack of LDH release ( Fig. 1b–d ). These patterns in cell toxicity were observed across multiple cell types, including MC3T3-E1 pre-osteoblasts, MB-MDA-231 breast cancer cells and primary human mesenchymal stem cells (hMSCs) ( Supplementary Fig. 4 ). The cell toxicity resulted from direct contact with the PA 1 nanofibre substrate. Any PA fragments that may be released into solution from the coating played a minimal role in cell death, as cells that were placed adjacent to PA 1 coatings with shared culture medium remained viable ( Supplementary Fig. 5 ). Additionally, when the assemblies were introduced in solution instead of being used as a coating, the cytotoxicity was conserved ( Supplementary Fig. 6 ). 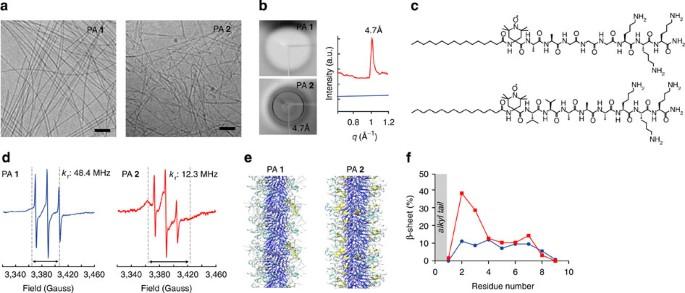Figure 2: Nanostructure and supramolecular cohesion within PA 1 and PA 2 assemblies. (a) Cryogenic TEM showing representative nanostructures in cell media. Scale bars, 100 nm. (b) X-ray diffraction of solutions of PA1(blue) and PA2(red). 4.7 Å corresponds to β-sheet hydrogen bonding. (c) Chemical structures of the spin-labelled analogues of PA1(top) and PA2(bottom) with a site-specific spin label (TOAC) located at the first amino acid adjacent to the fatty acid tail to probe the β-sheet hydrogen-bonding segment of the assemblies. (d) Electron paramagnetic resonance spectra of PA1and PA2combined with 20% of the corresponding spin-labelled analogue. Dashed lines and double-headed arrows indicate the spectral broadening that occurs with reduced rotational diffusion (kr). (e) Atomistic modelling of PA1and PA2demonstrating differences in β-sheet hydrogen bonding (yellow: β-sheet hydrogen bonding, cyan: β-turn, grey: random coil, blue: alkyl tail). (f) Data from modelling experiments to determine the distribution of β-sheet hydrogen bonding within assemblies of PA1(blue) and PA2(red) as a function of residue number from the alkyl tail. Figure 2: Nanostructure and supramolecular cohesion within PA 1 and PA 2 assemblies. ( a ) Cryogenic TEM showing representative nanostructures in cell media. Scale bars, 100 nm. ( b ) X-ray diffraction of solutions of PA 1 (blue) and PA 2 (red). 4.7 Å corresponds to β-sheet hydrogen bonding. ( c ) Chemical structures of the spin-labelled analogues of PA 1 (top) and PA 2 (bottom) with a site-specific spin label (TOAC) located at the first amino acid adjacent to the fatty acid tail to probe the β-sheet hydrogen-bonding segment of the assemblies. ( d ) Electron paramagnetic resonance spectra of PA 1 and PA 2 combined with 20% of the corresponding spin-labelled analogue. Dashed lines and double-headed arrows indicate the spectral broadening that occurs with reduced rotational diffusion ( k r ). ( e ) Atomistic modelling of PA 1 and PA 2 demonstrating differences in β-sheet hydrogen bonding (yellow: β-sheet hydrogen bonding, cyan: β-turn, grey: random coil, blue: alkyl tail). ( f ) Data from modelling experiments to determine the distribution of β-sheet hydrogen bonding within assemblies of PA 1 (blue) and PA 2 (red) as a function of residue number from the alkyl tail. Full size image We expected that the increased β-sheet hydrogen bonding of PA 2 nanofibres would strengthen the intermolecular cohesion. We use the term ‘intermolecular cohesion’ to describe the extent to which attractive forces among molecules stabilize the supramolecular units. Therefore, we hypothesize that the more cohesive fibres formed by PA 2 support cell viability. This led us to probe the internal order and conformational dynamics within the assemblies using synchrotron X-ray diffraction (XRD) and electron paramagnetic resonance (EPR) spectroscopy, respectively. XRD of a PA 1 solution revealed diffuse and amorphous scattering, whereas PA 2 exhibited a strong Bragg reflection at 4.7 Å ( Fig. 2b ), indicative of crystalline hydrogen bonding between two adjacent β-strands [29] . Increased β-sheet hydrogen bonding in assemblies of PA 2 was further confirmed by Fourier transform infrared spectroscopy ( Supplementary Fig. 7 ). EPR spectroscopy was performed to investigate if β-sheet hydrogen bonding constrained the molecular mobility in our system. EPR with site-directed spin labelling has been used to gain insight into the structure, local microenvironment, and dynamics of systems such as proteins, lipid bilayers, polymers and amyloid fibrils [30] , [31] , [32] , [33] . With the intent of capturing the mobility of PA assemblies in the region that participates in β-sheet hydrogen bonding, a site-specific TOAC spin label was added adjacent to the alkyl tail and used as a probe for EPR experiments ( Fig. 2c ). Slower motion of the spin label in nanostructures of PA 2 is apparent by both comparing the breadth of the spectra [34] ( Fig. 2d , double-headed arrows), and carrying out spectral simulations ( Supplementary Fig. 8 ). Rotational diffusion coefficients ( k r ) after fitting the EPR spectra using a non-linear least squares algorithm demonstrated that the motion adjacent to the spin label was nearly four times faster in the PA with weaker hydrogen bonding (PA 1 : 48.4 MHz, PA 2 : 12.3 MHz, respectively). This molecular level detail demonstrates that the reduced hydrogen bonding results in increased mobility of the individual molecules within the assembly. Atomistic simulations were also performed as previously described [35] and further corroborated our experimental data demonstrating increased hydrogen bonding in PA 2 as compared with PA 1 ( Fig. 2e,f ). As another approach to tailor intermolecular forces, an analogue of the cytotoxic PA 1 with a UV-polymerizable diacetylene tail was synthesized. As polymerization of diacetylene occurs via a topochemical reaction, it has been used to study the degree of packing within the PA nanofibre assemblies and their behaviour on mixing [36] , [37] , [38] . Coatings of the polymerized PA exhibited a substantial improvement in cell viability compared with untreated controls ( Supplementary Fig. 9 ), demonstrating the significance of intermolecular cohesion for cell viability. Traditional surfactants (for example, Triton X-100, sodium cholate and cetyl trimethylammonium bromide) are known to induce cell lysis by membrane disruption near their critical micelle concentrations [39] , [40] . Therefore, to investigate whether a difference in the aggregation behaviour between PA 1 and PA 2 could correlate to the cellular response, we estimated the critical aggregation concentration (CAC) in solution using a Nile Red assay ( Supplementary Fig. 10 ). In this assay, the CAC is characterized by a sharp transition in blue shift of the Nile Red probe. We observed that both PA 1 and PA 2 molecules have CAC values within the same order of magnitude. Moreover, the PA concentrations we used in our experiments are above the experimental CAC, suggesting that previous literature in surfactant cell toxicity does not predict the differences observed in PA-induced cytotoxicity. Interactions of liposomes with nanofibres The cationic and amphiphilic character of PA 1 , in combination with its tendency to induce cell death with rapid release of cytosolic LDH suggest that interactions with the cell membrane may be contributing to cell toxicity. To determine if the disruption of the lipid membrane was an underlying cause for the cytotoxicity, we created giant liposomes of egg phosphatidylcholine with cell-like dimensions on a glass surface. Time-lapse phase contrast microscopy revealed occasional fusion of the untreated liposomes over time as previously reported [41] ( Supplementary Movie 1 ); similar liposome behaviour was observed on treatment with PA 2 nanostructures. However, the addition of PA 1 destroyed liposomes within a few minutes, suggesting a strong interaction between the PA assemblies and liposomes ( Fig. 3a,b ; Supplementary Movies 2 and 3 ). This observation suggests that the weaker intermolecular cohesion of PA 1 assemblies is the factor that leads to cell death. 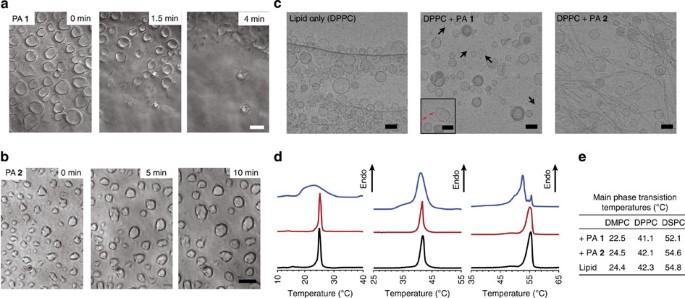Figure 3: Interactions between liposomes and peptide amphiphiles. Time-lapse phase contrast microscopy of giant liposomes exposed to either (a) PA1or (b) PA2. Time points are indicated in the upper right corner. Scale bars, 10 μm. (c) Cryogenic TEM of extruded DPPC liposomes (100 nm diameter) and mixtures with either molecule PA1or PA2. Inset: a less representative image of DPPC with PA1where a nanofibre is observed interacting with a liposome (black arrows: bicelles, red arrows: nanofibre). Scale bars, 100 nm. (d) Differential scanning calorimetry of liposome-PA1mixtures (blue), liposome-PA2mixtures (red) and liposomes alone (black) where the lipid component is comprised of DPPC (left), DMPC (middle) or DSPC (right). (e) Values of the gel-liquid crystalline phase transition temperatures from each DSC sample. Figure 3: Interactions between liposomes and peptide amphiphiles. Time-lapse phase contrast microscopy of giant liposomes exposed to either ( a ) PA 1 or ( b ) PA 2 . Time points are indicated in the upper right corner. Scale bars, 10 μm. ( c ) Cryogenic TEM of extruded DPPC liposomes (100 nm diameter) and mixtures with either molecule PA 1 or PA 2 . Inset: a less representative image of DPPC with PA 1 where a nanofibre is observed interacting with a liposome (black arrows: bicelles, red arrows: nanofibre). Scale bars, 100 nm. ( d ) Differential scanning calorimetry of liposome-PA 1 mixtures (blue), liposome-PA 2 mixtures (red) and liposomes alone (black) where the lipid component is comprised of DPPC (left), DMPC (middle) or DSPC (right). ( e ) Values of the gel-liquid crystalline phase transition temperatures from each DSC sample. Full size image The strong difference in the response of micron-sized liposomes to PA nanofibres prompted further investigations into PA–lipid interactions. To enable nanoscale characterization, liposomes of dipalmitoyl-phosphatidylcholine (DPPC) were extruded to a diameter of 100 nm and combined with assemblies of either PA 1 or PA 2 . We performed cryogenic transmission electron microscopy (cryoTEM) to evaluate structural changes following mixing. CryoTEM of DPPC mixed with assemblies of PA 1 compared with DPPC alone revealed drastic differences in liposome structure, including the presence of bicelles ( Fig. 3c , arrows) and irregularly shaped liposomes. Most of the high-aspect ratio nanostructures that were observed in solutions of PA 1 ( Fig. 2a ) were absent, suggesting their incorporation into the phospholipid component. In the few instances where nanofibres were observed, they were often associated with liposomes having irregular morphologies ( Fig. 3c , inset). In contrast, mixing DPPC with PA 2 nanofibres demonstrated the co-existence of both liposomes and fibres, suggesting that they interact less; moreover, the liposome morphologies were similar to those found with DPPC alone. Small-angle X-ray scattering corroborated these results, where liposome lamellarity was observed to change upon addition of PA 1 , but in the presence of PA 2 , no change was observed ( Supplementary Fig. 11 ). The disruption of both PA and liposome nanostructures in PA 1 –DPPC mixtures encouraged us to further evaluate changes in the lipid properties using differential scanning calorimetry (DSC) ( Fig. 3d ). DSC can monitor changes in the thermotropic properties of lipids and has been used previously to evaluate the ability of surfactants to self-organize separate from liposome assemblies [42] , [43] . DSC thermograms of either PA 1 or PA 2 alone had negligible signal ( Supplementary Fig. 12 ), thus the signal observed from the mixtures of PA and lipid can be attributed to the lipid component. When lipids with various tail lengths were mixed with the membrane-disrupting assemblies of PA 1 , both broadening and a shift in the gel to liquid-crystalline phase transition were observed ( Fig. 3d,e ). In contrast, the sharp phase transitions that were observed in the case of lipid alone were minimally perturbed in mixtures containing both liposomes and PA 2 assemblies. This result implies that PA 1 interacts with lipids more strongly, likely forming PA–lipid domains that alter the native thermal properties of the lipids. Furthermore, cryoTEM examination following thermal cycling from DSC experiments revealed negligible changes in the nanoscale morphology, thus eliminating the possibility that temperature was the contributing factor for the observed thermotropic properties ( Supplementary Fig. 13 ). These experiments suggest that the PA assemblies with reduced intermolecular cohesion disrupt the lipid component of a model phospholipid bilayer, whereas assemblies with increased cohesion remain intact and co-exist with liposomes. Interestingly, similar observations have been reported with amyloid fibrils, natural fibrillar aggregates of mis-folded proteins that are held together by β-sheet hydrogen bonding, where shorter fibrils have been shown to be more potent in disrupting model membranes as compared with their longer counterparts [44] . Although the authors attribute this result to increased free ends, our results suggest that intermolecular cohesion may also play a role in this phenomenon. Together, these experiments suggest that intermolecular cohesion may play a more general role in determining the ability of a supramolecular assembly to disrupt the phospholipid bilayer membrane. The role of membrane fluidity on cytotoxicity The composition of the cell membrane is complex and supported by an underlying cytoskeleton, thus we chose to determine if the interactions that we observed between PA and a model cell membrane translated to the native cell membrane. To examine the response of the cell membrane as it comes into contact with PA assemblies, MC3T3-E1 cell membranes were fluorescently labelled with a vital dye, DiI, and their viability was simultaneously monitored using calcein, a fluorescent dye that is retained within the cytoplasm by an intact cell membrane. The stained cells were allowed to settle on the PA-coated surfaces for about 5 min before imaging. Cells on coatings of PA 1 rapidly released calcein; in some cases, calcein release was preceded by an acute disruption to the cell membrane, which was identified as gaps in membrane continuity. ( Fig. 4a , arrows, Supplementary Movie 4 ). When the membrane dye was replaced with PA 1 containing a small fraction of its fluorescent analogue for visualization, PA 1 was found to localize strongly with the cell membrane. Moreover, occasional time-lapse images captured a brief period of membrane blebbing and calcein release, which occurred immediately before rupture. ( Fig. 4b , left and middle panels, Supplementary Movie 5 ). We speculate that the outer leaflet of the phospholipid bilayer is first populated with amphiphilic PA molecules or assemblies, which imparts local curvature strain, and initiates the catastrophic sequence of membrane blebbing and rupture [45] . However, a molecular dynamics simulation would be necessary to predict the exact molecular mechanism involved [46] . Although both PA 1 and PA 2 contain the same number of lysine residues, no co-localization of PA 2 with the cell membrane was observed above the focal plane of the PA coating ( Fig. 4b , right panel). We speculate that the reduced intermolecular hydrogen bonding in PA 1 enables dissociation of the assemblies from the coating surface, which associate with the dynamic plasma membrane, whereas PA 2 assemblies with the same formal charge as PA 1 assemblies are reinforced with hydrogen bonding, preventing separation from the nanofibre. Both PA assemblies concentrate charge locally on the nanostructure surface, however the propensity of PA 1 molecules to disassociate from the nanofibre may cause membrane disruption [46] . 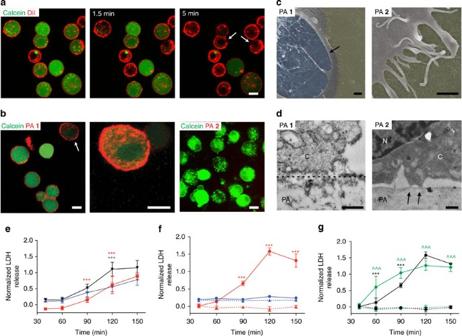Figure 4: Cell response to PA with varied β-sheet hydrogen bonding. (a) Confocal live cell imaging of cells treated with a membrane dye (DiI, red) and calcein (green) to visualize viability over time on coatings of PA1.Scale bar, 10 μm. Discontinuities in the cell membrane are indicated by arrows. (b) Confocal images of calcein-treated cells cultured on coatings of fluorescently labelled PA1(left) and higher magnification of the cell indicated by the arrow (centre). Calcein-treated cells cultured on coatings of fluorescently labelled PA2(right). Scale bars, 10 μm. (c) Scanning electron micrographs of cells on coatings of PA1and PA2after 30 min (yellow: coating surface, blue: internal surface of cell, no colour: outer cell surface). Scale bars, 500 nm. Arrow indicates the ruptured cell membrane. (d) Transmission electron micrographs of cross sections through both the cell and PA coating to reveal interactions between the cell and coating (C, cytoplasm; N, nucleus; PA, PA coating) after 30 min of culture (dashed line, interface between cell and PA coating; arrows, distinct sites of cell attachment to PA coating). Scale bars, 500 nm. (e–g) Time-dependent measurement of LDH release: (e) LDH release after inhibition of actin (blue) or myosin (red) were compared with untreated controls (black); (f) LDH release from cells cultured at either 37 °C (red) on coatings of PA1(circles, solid line) or PA2(triangles, dotted line). Cells were also cultured at 4 °C (blue) on PA1(circles, solid line) or PA2(triangles, dotted line); (g) LDH release from cells depleted of ATP (green) and cultured on coatings of PA1(solid line) or PA2(dotted line) were compared against control (black) cultures on PA1(solid line) or PA2(dotted line) coatings. Statistical analysis: two-way ANOVA with a Bonferroni post-test: ***P<0.001, treatments compared against their respective controls;P<0.001, PA1compared against PA2both with treatment. Figure 4: Cell response to PA with varied β-sheet hydrogen bonding. ( a ) Confocal live cell imaging of cells treated with a membrane dye (DiI, red) and calcein (green) to visualize viability over time on coatings of PA 1. Scale bar, 10 μm. Discontinuities in the cell membrane are indicated by arrows. ( b ) Confocal images of calcein-treated cells cultured on coatings of fluorescently labelled PA 1 (left) and higher magnification of the cell indicated by the arrow (centre). Calcein-treated cells cultured on coatings of fluorescently labelled PA 2 (right). Scale bars, 10 μm. ( c ) Scanning electron micrographs of cells on coatings of PA 1 and PA 2 after 30 min (yellow: coating surface, blue: internal surface of cell, no colour: outer cell surface). Scale bars, 500 nm. Arrow indicates the ruptured cell membrane. ( d ) Transmission electron micrographs of cross sections through both the cell and PA coating to reveal interactions between the cell and coating (C, cytoplasm; N, nucleus; PA, PA coating) after 30 min of culture (dashed line, interface between cell and PA coating; arrows, distinct sites of cell attachment to PA coating). Scale bars, 500 nm. ( e – g ) Time-dependent measurement of LDH release: ( e ) LDH release after inhibition of actin (blue) or myosin (red) were compared with untreated controls (black); ( f ) LDH release from cells cultured at either 37 °C (red) on coatings of PA 1 (circles, solid line) or PA 2 (triangles, dotted line). Cells were also cultured at 4 °C (blue) on PA 1 (circles, solid line) or PA 2 (triangles, dotted line); ( g ) LDH release from cells depleted of ATP (green) and cultured on coatings of PA 1 (solid line) or PA 2 (dotted line) were compared against control (black) cultures on PA 1 (solid line) or PA 2 (dotted line) coatings. Statistical analysis: two-way ANOVA with a Bonferroni post-test: *** P <0.001, treatments compared against their respective controls; P <0.001, PA 1 compared against PA 2 both with treatment. Full size image Electron microscopy further supported the findings from the experiments performed with model cell membranes and cells. Scanning electron microscopy (SEM) of cells exposed to a PA 1 coating for 30 min exhibited rough and irregular surfaces indicative of a severely compromised cell membrane, and in several cells, a clear rupture of the membrane was observed ( Fig. 4c ). Furthermore, when PA was added in soluble form, SEM revealed healthy, spread cells with intact assemblies of PA 2 on the membrane surface, showing that these assemblies interact with the cell membrane without toxicity, whereas assemblies of PA 1 resulted in irregular membrane surfaces similar to PA coatings ( Supplementary Fig. 14 ). TEM cross-sectional analysis of resin embedded samples with cells on PA 1 coatings revealed a poorly defined cell–material interface ( Fig. 4d , dotted line) with low amounts of electron dense material in the cytosol and abundant vacuole formation, suggestive of necrotic cell death. In contrast, cells on PA 2 had smooth membrane morphologies with active filopodial extensions at the periphery ( Fig. 4c ) and distinct contacts with the PA surface ( Fig. 4d , arrows), indicating minimal disturbance to the cell membrane. Although the cell response to the weakly cohesive PA is similar to the model liposomes, the inherent complexity of the cellular structures may introduce additional factors in the cell–nanostructure interaction. As actin polymerization and myosin activation are important during the initial phase of cell spreading and contribute to membrane tension [47] , we tested whether their inhibition could have an effect on the cell response to PAs. However, the inhibition caused no significant difference in the time-course for the release of the cytosolic enzyme LDH in comparison with controls ( Fig. 4e ; Supplementary Fig. 15 ). To test if membrane fluidity is critical for cell death, we performed experiments at reduced temperatures with the intent of slowing mobility. Compared with experiments performed at 37 °C, LDH release at 4 °C was markedly lower on PA 1 coatings ( P <0.001, two-way analysis of variance) and comparable to PA 2 controls (no significant difference between PA 1 and PA 2 at 4 °C), suggesting rescue of membrane disruption and cell death ( Fig. 4f ). However, reduced temperature is also known to slow metabolic processes, which may contribute to the observed effect. To test the influence of cell metabolic activity in the presence of PA, we depleted cells of ATP (~95% of total ATP activity; Supplementary Fig. 16 ) and exposed them to PA coatings. The ATP-depleted cells exhibited a similar LDH release profile as untreated samples (trends were similar to those in Fig. 1d ), suggesting that the interaction of PA and the cell membrane is independent of the metabolic state of the cell ( Fig. 4g ). Thus, cell death with weakly cohesive PA 1 nanofibres occurs through a biophysical process that is temperature-dependent, yet ATP-independent. Cell compartmentalization using cytotoxic nanostructures We next explored if the contact-mediated cytotoxicity of the weakly cohesive PA 1 could be exploited to contain cell migration in hydrogels. Although specific cell types cluster and segregate in tissues during processes such as organogenesis, wound healing and tumorigenesis, the ability to recapitulate this ordered cellular architecture in an artificial matrix is limited [48] , [49] . To this end, we sought to build a model three-dimensional microenvironment with two distinct niches that would allow free exchange of soluble factors but limit the migration of cells between the compartments. Two discrete hydrogel compartments with a coating of either PA 1 or PA 2 assemblies at the interface was created ( Fig. 5a,b ). We observed that cell viability inside the hydrogel was maintained in the presence of either PA coating. As expected, during sample preparation the PA 1 coating caused a small amount of cell death at the hydrogel periphery ( Fig. 5c ). During 1 week of culture, we observed that PA 1 preferentially prevented cell migration from one compartment to the other ( Fig. 5d , Supplementary Fig. 17 ). Moreover, cell nuclei were not found at the interface with PA 1 ( Fig. 5d , left panel), suggesting that cells were not constantly migrating to the interface and dying. Although the mechanism for containment is beyond the scope of this manuscript, we speculate that the biophysical phenomenon of membrane disruption may be occurring in localized regions of the cell membrane as the cell approaches the PA 1 coating. This localized damage of the membrane may act as a signal to prevent the migration across the toxic interface between the hydrogels. This result suggests that a coating of assemblies with weak cohesion can serve as a barrier to migrating cells and provide an approach to isolate cell populations while independently controlling their microenvironment. 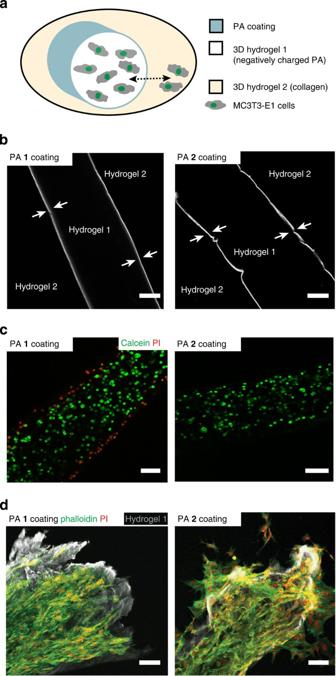Figure 5: Creating a cell barrier with PA coatings to compartmentalize cells. (a) A schematic of the experimental setup. A cell-encapsulated hydrogel (palmitoyl-VVAAEE 1%, w/v, hydrogel 1) is surrounded by collagen (hydrogel 2) with PA1or PA2coating at the interface. The experiment evaluates the cell migration through the hydrogel interface from hydrogel 1 to hydrogel 2 (dashed double-headed arrow). (b) A representative confocal slice from the two-compartment hydrogel system (as shown ina, but without cells) where hydrogel 1 is coated with either fluorescently labelled PA1or fluorescently labelled PA2(arrows indicate the coating layer which is ~10 μm thick). Scale bars, 100 μm. (c) Viability of MC3T3-E1 cells that were encapsulated in the hydrogel 1, coated with either PA1or PA2, and stained after 1 h with calcein (green, live cells) and propidium iodide (red, dead cells). Scale bars, 100 μm. (d) PA1- or PA2-coated cell encapsulating hydrogel 1 were further embedded in hydrogel 2 (as in the illustration ina) and cultured for 7 days, before staining for actin (phalloidin, green) and nuclei (propidium iodide, red). Cells remained confined within the hydrogel 1 compartment (grey) when coated with PA1, whereas cells escaped into the surrounding collagen when coating was done with PA2. Scale bars, 100 μm. Figure 5: Creating a cell barrier with PA coatings to compartmentalize cells. ( a ) A schematic of the experimental setup. A cell-encapsulated hydrogel (palmitoyl-VVAAEE 1%, w/v, hydrogel 1) is surrounded by collagen (hydrogel 2) with PA 1 or PA 2 coating at the interface. The experiment evaluates the cell migration through the hydrogel interface from hydrogel 1 to hydrogel 2 (dashed double-headed arrow). ( b ) A representative confocal slice from the two-compartment hydrogel system (as shown in a , but without cells) where hydrogel 1 is coated with either fluorescently labelled PA 1 or fluorescently labelled PA 2 (arrows indicate the coating layer which is ~10 μm thick). Scale bars, 100 μm. ( c ) Viability of MC3T3-E1 cells that were encapsulated in the hydrogel 1, coated with either PA 1 or PA 2 , and stained after 1 h with calcein (green, live cells) and propidium iodide (red, dead cells). Scale bars, 100 μm. ( d ) PA 1 - or PA 2 -coated cell encapsulating hydrogel 1 were further embedded in hydrogel 2 (as in the illustration in a ) and cultured for 7 days, before staining for actin (phalloidin, green) and nuclei (propidium iodide, red). Cells remained confined within the hydrogel 1 compartment (grey) when coated with PA 1 , whereas cells escaped into the surrounding collagen when coating was done with PA 2 . Scale bars, 100 μm. Full size image In summary, we have demonstrated here the strong impact of supramolecular cohesion in nanostructures to maintain cell membrane integrity and viability. Less cohesive assemblies were found to rapidly incorporate into the phospholipid bilayer, causing disruption of the cell membrane and contact-mediated cell death. Cell viability was rescued by increasing intermolecular cohesion within the nanostructure. Furthermore, we demonstrate the ability to create a material that can act as a barrier to cell migration in 3D culture. Intermolecular cohesion may have implications in toxicity of naturally occurring biological assemblies and provides guidelines for the design of nanostructured biomaterials that function to signal cells or deliver cargo. Peptide amphiphile synthesis PA molecules were synthesized using standard fluorenylmethyloxycarbonyl (Fmoc)-solid-phase peptide chemistry. The peptide segment and palmitic acid of molecules 1 – 11 were synthesized using a CEM Liberty microwave-assisted peptide synthesizer on Rink amide MBHA resin (Apptec) at the Peptide Synthesis Core at the Institute for BioNanotechnology in Medicine. Amino-acid couplings were performed with 5 equivalents (eq.) of protected amino acid or palmitic acid, 5 eq. of O -benzotriazole- N , N , N ′, N ′-tetramethyluronium hexafluorophosphate (HBTU) and 10 eq. of N , N -diisopropylethylamine (DIEA) at 75 °C for 5–10 min. Fmoc deprotection was performed using 20% 4-methyl piperidine and 0.1 M hydroxybenzotriazole (HOBt) in dimethylformamide (DMF) at 75 °C for 3–4 min. Capping steps were achieved using a mixture of 0.5 M acetic anhydride, 0.125 M DIEA and 0.015 M HOBt in DMF at 65 °C for 2 min. Default microwave settings were used. The alkyl tails were coupled using 4 eq. of dodecanoic, myristic or eicosanoic acid (Sigma-Aldrich) with 3.95 eq. of HBTU and 6 eq. DIEA in a solvent mixture of 1:1:1 DMF:dichloromethane (DCM): N- methyl-2-pyrrolidone (NMP) for 3–4 h. ( Supplementary Figs 18 and 19 ). Fluorescent molecules were synthesized ( Supplementary Figs 20 and 21 ) using Universal Novatag resin (EMD Chemicals). Deprotection of the monomethoxytrityl (Mmt)-protecting group was performed with 0.6 M N -hydroxybenzotriazole in 1:1 trifluoroethanol:DCM for 30 min. The fluorophore was coupled with 1.1 eq. 5(6)-carboxy-tetramethylrhodamine (EMD Chemicals), 1.1 eq. PyBOP and 2.2 eq. DIEA in DMF overnight. PA molecules 10 and 11 contain a nitroxide spin radical for EPR ( Supplementary Fig. 22 ). Fmoc-TOAC, an unnatural amino acid, which was synthesized as previously described [50] replaced the first amino acid adjacent to the alkyl tail. The spin-labelled amino acid Fmoc-TOAC was coupled using 2.5 eq. of Fmoc-TOAC, 2.45 eq. of HBTU, and 6 eq. of DIEA in NMP. To couple the UV-polymerizable tail to PA molecule 12 , 2 eq. of 10,12-pentacosadiynoic acid (Fluka), 1.95 eq. of HBTU and 3 eq. of DIEA in a solvent mixture of 1:1:1 DMF:DCM:NMP was added overnight and protected from light. Following synthesis, molecules were cleaved in a mixture of 95:2.5:2.5 trifluoroacetic acid:triisopropylsilane:water for 2–3 h. The solvent was removed using rotary evaporation and the product was precipitated using cold diethyl ether. The product was dried under vacuum over a frit and purified by preparative scale reverse-phase high-performance liquid chromatography using a Phenomenex Jupiter Proteo column (C 12 stationary phase, 10 μm, 90 Å pore size, 30 × 150 mm) for molecules 1 – 6 and 8 – 12 or a Phenomenex Gemini column (C 18 stationary phase, 5 μm, 100 Å pore size, 30 × 150 mm) for molecule 7 with a gradient of acetonitrile and water containing 0.1% TFA (Jupiter) or 0.1% NH 4 OH (Gemini). Pure fractions were identified using ESI mass spectrometry, collected, subjected to rotary evaporation to remove excess acetonitrile, lyophilized and stored at −20 °C until use. Analytical HPLC was performed using an Agilent 6520 QTOF-LCMS with similar Phenomenex columns. X-ray diffraction Wide-angle X-ray diffraction was performed using a bending magnet station (14-BMC, Argonne National Laboratory, Argonne, IL). All data were obtained at 12.67 keV (wavelength: 0.979 Å). Samples were dissolved to 1% (w/v) in a 1:1 mixture of water:MEM-Alpha and injected into 1.5-mm diameter quartz capillaries (Charles Supper). The capillaries were held in place using moudling clay fitted to a magnetic mount. Scattering from the solvent alone was used as background. Background solvent subtraction and radial integration were performed using FIT2D software. Cryogenic transmission electron microscopy CryoTEM was performed using a JEOL 1230 TEM fitted with a LaB 6 filament working at an accelerating voltage of 100 kV. Samples were plunge frozen using a Vitrobot Mark IV (FEI) vitrification robot operating at 21 °C with 100% humidity. The sample (5 μl) was deposited on a 300-mesh copper grid (Electron Microscopy Sciences, EMS) with lacey carbon support, blotted and plunged into a liquid ethane reservoir cooled by liquid nitrogen. Following vitrification, the sample was transferred under liquid nitrogen to a Gatan 626 cryo-holder. Images were acquired using a Gatan 831 CCD camera. PAs were imaged at 0.05–0.1% (w/v) in a 1:1 mixture of water:MEM-Alpha media. Mixtures of molecules 1 and 2 mixed with 20% (v/v) of their spin-labelled analogues were imaged at 0.1% (w/v) in 0.5 × PBS buffer to maintain consistency with EPR experiments. Extruded DPPC liposomes were imaged at 5 mM in 0.5 × PBS buffer (1.3 mM KCl, 0.74 mM KH 2 PO 4 , 68.97 mM NaCl, 4.03 mM Na 2 HPO 4 ) and DPPC PA mixtures were imaged with 5 mM DPPC+1 mM PA in 0.5 × PBS. Nile Red assay The self-assembly of the PAs was assessed by incorporation of the hydrophobic solvatochromic probe Nile Red (9-diethylamino-5-benzo[α]phenoxazinone), which exhibits an emission blue shift on inclusion in hydrophobic environments [51] , [52] . Solutions of molecules 1 and 2 , ranging from 1 μM to 1,000 μM in PBS, were prepared from stock solutions, and Nile Red in ethanol was diluted 200-fold into solutions to a final concentration of 250 nM. Using a NanoLogHJ spectrofluorometer, the samples were excited at 550 nm and the spectra were collected from 580–750 nm. Blue shifts were calculated by subtracting the emission wavelength of the sample from the emission wavelength of Nile Red in PBS and were plotted against concentration to determine the critical aggregation concentrations.. PA coatings Forty-eight-well tissue-culture-treated plates or glass coverslips were coated with 0.01% (w/v) poly- D -lysine (PDL, Sigma-Aldrich) diluted in a borate buffer for a minimum of 1 h at room temperature (RT). These coatings were then washed three times with sterile water followed by a second coating of 0.25% (w/v) sodium alginate (FMC Biopolymer) solution in water for 1 h at RT. Excess solution was removed and 10 mM CaCl 2 was added to make a thin layer of alginate gel. 0.01–0.05% (w/v) PA diluted in 2 mM CaCl 2 was added on top of the alginate layer, incubated overnight at 37 °C and washed two times with MEM-Alpha before performing experiments. For time-lapse experiments, coatings were performed as described above on glass-bottom Petri dishes. Fluorescent PA was coated at a concentration of 1:100 fluorescent PA: non-fluorescent PA for coatings. To assess cell viability and visualize the cell membrane, the cells were incubated for 15 min at 37 °C in serum-free media containing 5 μl ml −1 DiI (Invitrogen) and/or 5 μl ml −1 calcein (Invitrogen). Cells were centrifuged and washed three times with media and added directly to the coatings for imaging. Time-lapse images were recorded using a Zeiss LSM 510 META confocal microscope. Cell culture MC3T3-E1 subclone 4 pre-osteoblast cells (ATCC) passages 3–10 were maintained in growth media containing MEM-Alpha medium (Invitrogen) supplemented with 10% heat-inactivated fetal bovine serum (HI-FBS, Invitrogen), 50 U ml −1 penicillin and 50 μg ml −1 streptomycin (P/S, Invitrogen). MB-MDA-231 breast cancer cells (ATCC) passages 20–30 were maintained in high-glucose DMEM (Invitrogen) supplemented with 10% HI-FBS, 50 U ml −1 50 μg ml −1 P/S. hMSCs (Lonza) passages 2–5 were cultured using hMSC growth media (Lonza). Cells were cultured until 80–90% confluence, passaged using 0.05% Trypsin/EDTA (Invitrogen) and seeded for experiments. To assess cell viability, 20,000 cells were incubated on the PA coatings in serum-free MEM-Alpha for 4–5 h either in a 48-well plate or on 12-mm-coated glass coverslips. Cells were then exposed to calcein AM (Invitrogen) and ethidium homodimer-1 (Invitrogen) following manufacturer’s protocols. Stained cells were imaged using an inverted fluorescent microscope (Nikon, Eclipse TE2000U). For experiments with shared culture media,glass coverslips were adhered to a 60-mm tissue culture plastic dish using non-toxic vacuum grease and cells were cultured for 4 h with shared media before viability staining. For LDH release, cells were seeded at 30,000 cells per well in a 48-well plate in triplicate and enzyme release was measured using the CytoTox 96 non-radioactive cytotoxicity assay (Promega) following the manufacturer’s protocol. Phenol-free MEM-Alpha (Invitrogen) was used to seed the cells on the coatings and the media was sampled at desired time points and normalized with a 1% Triton X-100-treated positive control, which represented 100% LDH release. For ATP-depletion experiments, cells were incubated in serum-free media containing 0.1% NaN 3 and 50 mM 2-deoxy- D -glucose (Sigma-Aldrich). Inhibition of myosin II activity was achieved with 0.05 mM blebbistatin (Calbiochem) and inhibition of actin polymerization was performed with 500 nM latrunculin A (Calbiochem). For the ATP-depletion and cytoskeletal inhibition studies, adherent cells were treated in serum-free media for 1 h at 37 °C. Following treatment, cells were trypsinized and added to PA coatings in serum-free MEM-Alpha with the respective additives. For cell-barrier (compartmentalization) experiments, the desired number of cells were centrifuged into a pellet, resuspended in a small volume of media and further resuspended in a solution of a negatively charged PA molecule (palmitoyl-Val-Val-Ala-Ala-Glu-Glu) that was previously thermally annealed to 80 °C for 30 min to aid with gel formation. This yielded a final PA concentration of 0.75% (w/v) and a final cell concentration that ranged from 10,000 to 100,000 cells per μl. The PA solution with suspended cells was then drawn into a gelling solution containing 10 mM CaCl 2 , 132 mM NaCl and 3 mM KCl to make a cylindrically shaped gel, which was then broken into short pieces, immersed for 1 min in a solution containing 0.01% (w/v) of either PA 1 or PA 2 in a solution of 147 mM NaCl and 3 mM KCl. The gels were then rinsed three times in PBS and were encapsulated in a 2.5 mg ml −1 collagen gel (rat tail, type I; BD) using a glass-bottom Petri dish (Mattek). Cells were cultured then fixed with 4% paraformaldehyde, permeabilized with 0.4% Triton X-100, and stained with propidium iodide (500 ng ml −1 , Sigma-Aldrich) to visualize nuclei and phalloidin-Alexa Fluor 488 (1:100 dilution, Invitrogen) to visualize F-actin. DAPI staining (5 μg ml −1 , Invitrogen) aided with visualization of the PA gel, as a high degree of non-specific binding to the negatively charged PA was consistently observed. Statistical analysis and image analysis All results are presented as the mean±s.d. All experiments were performed with a minimum of three independent runs and statistical analysis was performed using Prism. Cell viability on different PA coatings was evaluated using a one-way ANOVA with a Tukey post-hoc test and compared with PA 2 , the non-toxic PA coating. The LDH release data was analysed using a two-way ANOVA with a Bonferroni post-test to assess differences between groups at each timepoint. A value of P <0.001 was considered to be significant. Processing of images obtained from fluorescent and phase microscopy were performed using NIH Image J. Gamma values of all images maintained at 1 and only linear manipulations of brightness and contrast were performed. Giant liposome experiments Giant liposomes were prepared on a surface to enable time-lapse microscopy as described previously [41] . One side of a glass slide was dipped into melted agarose (low-melting temperature, Amresco). Excess agarose solution was removed and the glass slide was placed on a 45 °C hot plate until dry. Egg phosphatidylcholine (Sigma-Aldrich) was dissolved at 3.75 mg ml −1 in chloroform and a total of 30 μl was added dropwise to the agarose film and quickly rolled across the glass slide using a pasteur pipet. Samples were incubated under vacuum overnight to remove residual solvent, followed by hydration of the lipid films with PBS. PA was added to the hydrated liposomes at a final concentration of 0.2% (w/v) and monitored using time-lapse phase contrast images (Nikon, Eclipse TE2000U). As a control, PBS without PA was added to confirm that changes in osmolarity were not playing a dominant role; in this control, no significant changes were observed. Extruded liposome experiments Liposomes of ~100 nm diameter were prepared by extrusion. Briefly, DPPC (Avanti Polar Lipids) was dissolved in chloroform to a concentration of 10 mM and dried to a film using rotary evaporation. The films were maintained under vacuum overnight to remove any excess solvent. Dried films were hydrated with buffer (1.3 mM KCl, 0.74 mM KH 2 PO 4 , 68.97 mM NaCl, 4.03 mM Na 2 HPO 4 ) to a concentration of 10 mM at 60 °C before performing 4–5 freeze thaw cycles to improve unilamellarity of the liposomes. The hydrated lipid solution was then extruded 15 times through a 100-nm-pore-size polycarbonate filter (Whatman) using an Avanti mini-extruder at 60 °C to maintain membrane fluidity. For mixing experiments, PA solutions were dissolved in water at 10 mM and diluted to match the solvent used for lipid extrusion. The final mixtures contained 5 mM DPPC and 1 mM PA. Differential scanning calorimetry DSC thermograms were obtained using a MicroCal VP-DSC with high feedback gain and filtering period of 1 s. Data from the heating cycles were reported, as suggested by the manufacturer. Heating and cooling cycles were performed at 1 °C per min from 20 °C to 60 °C for DPPC, 30 °C to 80 °C for DSPC (Avanti Polar Lipids), and 5 °C to 40 °C for DMPC (Avanti Polar Lipids) until thermograms for the heating and cooling cycles matched, suggesting that thermodynamic equilibrium was reached. Lipids were extruded through 100-nm-pore track etch membranes before mixing with PA for a final concentration of 2.5 mM lipid and 1 mM PA. Thermograms of lipid alone were performed at a concentration of 2.5 mM. Scanning electron microscopy For performing SEM, coatings were made on glass coverslips (EMS) as described above. Cells were allowed to settle on coatings for 30 min and fixed immediately with 2.5% glutaraldehyde in PBS for 1 h at RT. The samples were then dehydrated using a gradient from water to ethanol until samples were immersed in 100% ethyl alcohol and dried at the critical point of CO 2 using a critical point dryer (Tousmis Samdri-795) to preserve structure. Samples were then coated with 12 nm of osmium metal using an osmium plasma coater (Filgen, OPC-60 A) and imaged using a Hitachi S-4800 FE-SEM secondary electron detector with an accelerating voltage of 5 kV. Transmission electron microscopy PA coatings were made on glass coverslips and cells were allowed to adhere on the coatings for 30 min before primary fixation (2% glutaraldehyde, 2% paraformaldehyde in 0.1 M cacodylate buffer, 1 mM CaCl 2 , pH 7.4) for 1 h. Samples were post-fixed (2% osmium tetroxide in cacodylate) for 2 h at RT, followed by an en-block stain (3% uranyl acetate) for 1 h on ice. The sample was then dehydrated with a graded series of ethanol to 100% ethyl alcohol, infiltrated with Epon 812 resin (EMS) over 2 days, and cured at 60 °C overnight in flat embedding moulds. The glass coverslip was dissolved using concentrated hydrofluoric acid and sectioning was performed using a Leica Ultracut S microtome. Images were acquired on a JEOL 1230 TEM operating at 80 kV. Electron paramagnetic resonance EPR spectroscopy was performed using a modified Varian E-4 with a 9.8 GHz frequency with a 200 Gauss sweep width. Modulation amplitudes were maintained below 0.2 times the peak-to-peak line widths. Samples were injected (3–5 μl) into PTFE capillary tubing (outer diameter, 0.8 mm), sealed using Critoseal sealant, and placed in a quartz EPR tube. Samples were inserted into a rectangular resonator cavity and spectra were collected at RT. Each PA was mixed with the 20% (v/v) spin-labelled analogue and measured at 0.1% (w/v) in buffer (0.5 × PBS). Spectral simulations were performed using a non-linear least squares analysis via the Levenberg–Marquardt algorithm (Acert software package). A total of 13 parameters were varied, including the rotational coefficient (rbar), which was extracted and used to derive the rotational diffusion rate ( k r ) given the equation 10 rbar = k r . All spectral fits obtained had correlation values above 98%. Atomistic modelling The starting structure of each PA was assumed to be in an extended conformation. To define an initial fibre structure, nine PAs were radially placed on a plane with the tails pointing inward. The angle between adjacent PAs was 40°. The second layer was identical to the first layer but rotated by 20° relative to the first layer and the distance between layers was set to 5 Å. A total of 14 layers that alternate between the first and second layers were placed along the fibre axis to define the complete structure. A total of 126 PA molecules (14 × 9=126) were solvated in a water box using the SOLVATE [53] module implemented in VMD [54] . Periodic boundary conditions using a box of dimensions of 122 × 122 × 64 Å 3 filled with 22,669 (for PA 1 ) or 22,285 (for PA 2 ) water molecules was used (based on the modified TIP3P potential) [55] , [56] . To neutralize the system, 378 Cl – ions were added with an additional 65 Na + and Cl – ions to provide a final concentration of 150 mM NaCl. A 1,000-step energy minimization was applied to the solvated system to remove the high-energy contacts. Molecular dynamics simulations were carried out using NAMD2 (ref. 57 ) A 1-ns molecular dynamics simulation at 800 K with a NVT ensemble was performed to equilibrate the system. During the equilibration, the positions of tails are fixed to avoid the dissipation of PA molecules. In the production period, the system was simulated for 16 ns using the NPT ensemble and Langevin dynamics [58] at a temperature of 310 K with a damping coefficient γ =5 ps –1 . Pressure was maintained at 1 atm using the Langevin piston method with a piston period of 100 fs, a damping time constant of 50 fs and piston temperature of 310 K (refs 58 , 59 ). No atomic coordinates were constrained during the production period. Full electrostatics was employed using the particle-mesh Ewald method with a 1-Å grid width [60] . Non-bonded interactions were calculated using a group-based cutoff with a switching function and were updated every ten time steps. Covalent bonds involving hydrogen were held rigid using the SHAKE algorithm [61] , allowing a 2-fs time step. Atomic coordinates were saved every 10 ps for the trajectory analysis. How to cite this article: Newcomb, C. J. et al. Cell death versus cell survival instructed by supramolecular cohesion of nanostructures. Nat. Commun. 5:3321 doi: 10.1038/ncomms4321 (2014).